Ubiquitination and degradation of the FADD adaptor protein regulate death receptor-mediated apoptosis and necroptosis Fas-associated protein with death domain (FADD) is a pivotal component of death receptor-mediated extrinsic apoptosis and necroptosis. Here we show that FADD is regulated by Makorin Ring Finger Protein 1 (MKRN1) E3 ligase-mediated ubiquitination and proteasomal degradation. MKRN1 knockdown results in FADD protein stabilization and formation of the rapid death-inducing signalling complex, which causes hypersensitivity to extrinsic apoptosis by facilitating caspase-8 and caspase-3 cleavage in response to death signals. We also show that MKRN1 and FADD are involved in the regulation of necrosome formation and necroptosis upon caspase inhibition. Downregulation of MKRN1 results in severe defects of tumour growth upon tumour necrosis factor-related apoptosis-inducing ligand treatment in a xenograft model using MDA-MB-231 breast cancer cells. Suppression of tumour growth by MKRN1 depletion is relieved by simultaneous FADD knockdown. Our data reveal a novel mechanism by which fas-associated protein with death domain is regulated via an ubiquitination-induced degradation pathway. Apoptosis, or programmed cell death, can be initiated by intrinsic or extrinsic pathways [1] , [2] . Intrinsic pathways are triggered by mitochondrial permeabilization, which results in the release of cytochrome c and the formation of an apoptosome complex, leading to caspase-9 activation [3] . Extrinsic pathways can be induced by activation of death receptors (DRs), such as TNFR1, tumour necrosis factor-related apoptosis-inducing ligand (TRAIL) receptors and Fas/CD95 by their corresponding ligands; receptor activation triggers the formation of the death-inducing signalling complex (DISC) or TNFR complex II, which comprises caspase-8 and fas-associated protein with death domain (FADD). These complexes ultimately activate caspase-8, thereby causing extrinsic apoptosis [3] , [4] . In addition to inducing extrinsic apoptosis, caspase-8 and FADD are known to suppress necroptosis under various conditions [5] , [6] , [7] , [8] , [9] , [10] , [11] . DR downstream pathways are regulated in various ways. For example, cFLIP (cellular FLICE inhibitory protein) competes with caspase-8 for binding to FADD, preventing DISC formation [12] . The levels and activities of cFLIP are controlled by numerous factors including NF-κB, Akt, JNK, Srk and ITCH [13] , [14] , [15] , [16] , [17] . CARP-1 and -2, which are E3 ubiquitin ligases for caspase-8, are also known to suppress TRAIL activation [18] . Post-translational modifications such as O -glycosylation, S -nitrosylation and S -palmitoylation of DRs have also been identified to regulate death signalling [19] . However, phosphorylation of FADD, the only post-translational modification that FADD is known to undergo, is not involved in the induction of apoptosis. Rather, this modification seems to be essential for the pro-survival roles of nuclear-localized phospho-FADD [20] , [21] , [22] , [23] . Other post-translational modifications affecting the apoptotic and necroptotic activities of FADD have yet to be identified. Here, we show that Makorin Ring Finger Protein 1 (MKRN1), an E3 ligase involved in p53 and p21 regulation [24] , is able to induce ubiquitination-dependent degradation of FADD. Upon depletion of MKRN1, the protein level of FADD increased significantly, stimulating the formation of DR complexes for apoptosis. The association of MKRN1 and FADD also affected the process of necroptosis in such a way as to regulate drastic cell death. Using orthotropic xenograft tumour formation, we showed that MKRN1-depleted tumours are much more sensitive to TRAIL injection, implicating MKRN1 as a possible therapeutic target in cancer treatment. Finally, we found that the TRAIL sensitivity of MKRN1-depleted tumours was diminished by simultaneous FADD knockdown, indicating a critical link between these two proteins in cell death pathways. Depletion of MKRN1 induces DR-mediated extrinsic apoptosis MKRN1, a protein highly conserved from invertebrates to vertebrates, has a ubiquitous expression pattern in various tissues [25] and functions as an E3 ubiquitin ligase for various substrates [24] , [26] , [27] . Previous reports showed that MKRN1 was able to suppress p53 function, and regulate cell growth and apoptosis. Interestingly, we found that MKRN1 ablation in HeLa cells, in which p53 is suppressed by E6-mediated degradation, induced cell death as measured by the percentage of the subG1 fraction ( Fig. 1a ; Supplementary Fig. S1a,b ). Similar effects were detected in other p53-defective cell lines including H1299 and HCT116 p53−/−, as well as in p53-positive cell lines ( Supplementary Fig. S2 ). Here, p53 null cells were less affected by MKRN1 depletion than wild-type (WT) p53 cells. Annexin V/7-AAD double-staining analyses further verified that MKRN1 depletion increased early apoptosis ( Fig. 1b ; Supplementary Fig. S1c ). Treatment of HeLa cells with zVAD-fmk, a pan-caspase inhibitor, completely abrogated the effect of MKRN1 depletion on cell death, suggesting the involvement of MKRN1 in caspase-dependent apoptosis ( Fig. 1a,b ). To determine whether DR-mediated cell death pathways were involved, we measured the levels of cleaved-caspase-8 or -9. Cleaved-caspase-8 was detected after 72 h upon MKRN1 knockdown, while cleaved-caspase-9 was visualized after 96 h ( Fig. 1c ). To clarify which caspase was responsible for the initiation of the death pathway in detail, we treated cells with specific inhibitors for caspase-8, or -9. Inhibition of caspase-8 mostly prevented caspase-9 cleavage, while caspase-9 inhibition did not affect caspase-8 cleavage upon MKRN1 depletion ( Fig. 1d ). These results suggest that MKRN1 depletion presumably induces the caspase-8-dependent extrinsic apoptotic pathway by prompting caspase-8 activation, subsequently leading to caspase-9 and caspase-3 cleavage and apoptosis. Overall, these data suggest that MKRN1 knockdown induces a p53-independent extrinsic apoptotic process. 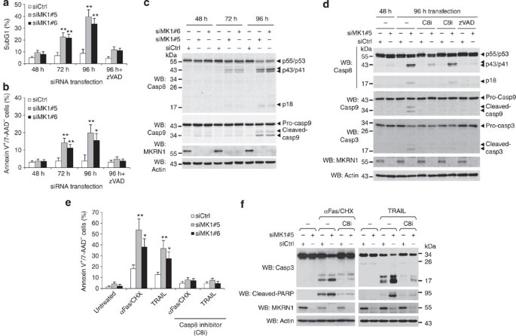Figure 1: MKRN1 knockdown induces caspase-8-dependent apoptosis. (a) HeLa cells were transfected with 20 nM of control siRNA (siCtrl) or two kinds of MKRN1 siRNA (siMK1#5, siMK1#6), and 20 μM zVAD (z-VAD-fmk) was added 24 h after transfection. Cells were harvested at 48, 72 and 96 h post transfection, stained with PI and analysed by flow cytometry. The data are presented inSupplementary Fig. S1band summarized ina(data are means±s.d.;n=3, **P<0.01 compared with siCtrl). (b) HeLa cells, transfected and treated with zVAD as described above, were harvested, immediately stained with Annexin V and 7-AAD, and analysed by flow cytometry. Dot plot data are shown inSupplementary Fig. S1c, and the Annexin V-positive/7-AAD-negative fraction percentages are shown inb(data are means±s.d.;n=3, *P<0.05, **P<0.01 compared with siCtrl). (c) HeLa cells were transfected with control siRNA (siCtrl) or MKRN1 siRNA (siMK1#5 or siMK1#6). Cells were harvested at 48, 72 and 96 h post transfection, lysed and immunoblotted with antibodies against casp8 (caspase-8), casp9 (caspase-9), MKRN1 and actin. (d) At 24 h after transfection, HeLa cells were treated with 20 μM of C8i (caspase-8 inhibitor, z-IETD-fmk), C9i (caspase-9 inhibitor, z-LEHD-fmk) and zVAD (pan-caspase inhibitor). Cells were harvested at 48 and 96 h post transfection and WB analysis using the indicated antibodies was performed. (e) HeLa cells, transfected with 20 nM of the indicated siRNAs, were treated with 50 ng ml−1anti-Fas antibody (αFas) plus 5 μg ml−1CHX or 100 ng ml−1TRAIL alone for 3 h in the absence or presence of 20 μM caspase-8 inhibitor. Cells were harvested, and Annexin V staining was conducted. The data are presented inSupplementary Fig. S5aand summarized ine(data are means±s.d.;n=3, *P<0.05, **P<0.01 compared with siCtrl). (f) HeLa cells, transfected with the indicated siRNAs, were pre-treated with C8i and stimulated with αFas or TRAIL. Apoptosis was determined by WB analysis using anti-Casp3 and anti-PARP antibodies. Figure 1: MKRN1 knockdown induces caspase-8-dependent apoptosis. ( a ) HeLa cells were transfected with 20 nM of control siRNA (siCtrl) or two kinds of MKRN1 siRNA (siMK1#5, siMK1#6), and 20 μM zVAD (z-VAD-fmk) was added 24 h after transfection. Cells were harvested at 48, 72 and 96 h post transfection, stained with PI and analysed by flow cytometry. The data are presented in Supplementary Fig. S1b and summarized in a (data are means±s.d. ; n =3, ** P <0.01 compared with siCtrl). ( b ) HeLa cells, transfected and treated with zVAD as described above, were harvested, immediately stained with Annexin V and 7-AAD, and analysed by flow cytometry. Dot plot data are shown in Supplementary Fig. S1c , and the Annexin V-positive/7-AAD-negative fraction percentages are shown in b (data are means±s.d. ; n =3, * P <0.05, ** P <0.01 compared with siCtrl). ( c ) HeLa cells were transfected with control siRNA (siCtrl) or MKRN1 siRNA (siMK1#5 or siMK1#6). Cells were harvested at 48, 72 and 96 h post transfection, lysed and immunoblotted with antibodies against casp8 (caspase-8), casp9 (caspase-9), MKRN1 and actin. ( d ) At 24 h after transfection, HeLa cells were treated with 20 μM of C8i (caspase-8 inhibitor, z-IETD-fmk), C9i (caspase-9 inhibitor, z-LEHD-fmk) and zVAD (pan-caspase inhibitor). Cells were harvested at 48 and 96 h post transfection and WB analysis using the indicated antibodies was performed. ( e ) HeLa cells, transfected with 20 nM of the indicated siRNAs, were treated with 50 ng ml −1 anti-Fas antibody (αFas) plus 5 μg ml −1 CHX or 100 ng ml −1 TRAIL alone for 3 h in the absence or presence of 20 μM caspase-8 inhibitor. Cells were harvested, and Annexin V staining was conducted. The data are presented in Supplementary Fig. S5a and summarized in e (data are means±s.d. ; n =3, * P <0.05, ** P <0.01 compared with siCtrl). ( f ) HeLa cells, transfected with the indicated siRNAs, were pre-treated with C8i and stimulated with αFas or TRAIL. Apoptosis was determined by WB analysis using anti-Casp3 and anti-PARP antibodies. Full size image As MKRN1 depletion initiated caspase-8 activation, we investigated the association between MKRN1 and DRs, such as Fas, DR4/5 and TNFR. First, kinetic treatment of HeLa cells with anti-Fas or TRAIL revealed that MKRN1 knockdown accelerated cell death compared with the control ( Supplementary Fig. S3a,b ). Treatment of cells with anti-Fas or TRAIL for 3 h significantly altered the morphology of the HeLa cells when MKRN1 was depleted, while control small interfering RNA (siRNA)-transfected cells displayed few changes. When cell death was enhanced by treatment with cycloheximide (CHX), a translation inhibitor, MKRN1 depletion resulted in severe cell death upon anti-Fas and TRAIL treatment compared with control cells ( Supplementary Fig. S4a,b ). In cells in which MKRN1 was ablated, anti-Fas- or TRAIL-dependent cell death was efficiently blocked by zVAD-fmk and a caspase-8 inhibitor, but not by necrostatin-1 (nec-1), a necroptosis inhibitor ( Supplementary Fig. S4a–c ) [20] , [28] , [29] . These results allowed us to eliminate the possible involvement of necroptosis. Furthermore, western blot (WB) analyses and annexin V/7-AAD staining indicated that MKRN1 depletion followed by stimulation with anti-Fas or TRAIL promoted caspase-3/PARP cleavage and apoptotic cell death, both of which were blocked by caspase-8 inhibitor ( Fig. 1e,f ). Next, we investigated whether MKRN1 affects DISC formation and subsequent caspase-8 activation. Upon MKRN1 depletion, caspase-8 cleavage occurred within 1 or 2 h after anti-Fas or TRAIL treatment, while it took 3 h in control cells ( Fig. 2a,b ). In accordance with this, we observed increased caspase-9 and caspase-3 cleavage as well as cell death upon DR activation in MKRN1-knockdown cells ( Supplementary Fig. S5 ). Upon caspase-8 inhibition, the cleavage of both caspase-9 and caspase-3 was prevented, implying a critical role for caspase-8 in DR-mediated apoptosis. Caspase-9 inhibition also ameliorated cell death in MKRN1-depleted cells upon DR activation despite caspase-8 cleavage, indicating that caspase-9 activity is also required for full apoptosis induction ( Supplementary Fig. S5b,c ). Based on these results, we immunoprecipitated DISC complexes at time points ranging from 0 to 2 h using control or MKRN1-depleted HeLa cells after anti-Fas or TRAIL treatment, followed by DISC-IP (immunoprecipitation) analysis. DISC complexes began to appear in MKRN1-depleted cells within 1 h, whereas DISC complexes were only detected after 2 h in control cells ( Supplementary Fig. S6a–c ). We also performed DISC analysis using a suspension of cells treated with higher concentrations of anti-Fas or TRAIL, which leads to faster DISC complex formation compared with the aforementioned methods [30] . Under these conditions, we also observed an increase in FADD–caspase-8–caspase-10 complex formation in MKRN1-depleted cells within 15 min when compared with the control ( Fig. 2c,d ). In addition, the recruitment of FLIP to DISC complexes was slightly increased ( Fig. 2c,d ). These results imply that DISC formation and caspase-8-mediated apoptosis are expedited by MKRN1 depletion. 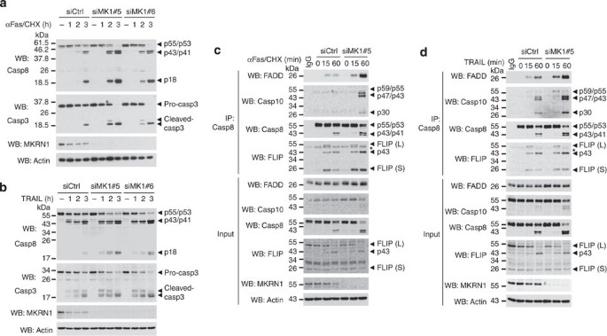Figure 2: MKRN1 depletion facilitates caspase-8 cleavage upon DR activation by causing rapid assembly of the DISC complex. (a,b) HeLa cells, transfected with the indicated siRNAs, were treated with 50 ng ml−1of αFas and 5 μg ml−1of CHX (a) or 50 ng ml−1of TRAIL (b) for 1–3 h as indicated. Lysates were immunoblotted with anti-Casp8 and anti-Casp3 antibodies. (c,d) HeLa cells, transfected with siRNAs, were harvested using trypsin at 48 h post transfection. Cells were resuspended in 1 ml of complete media and treated with 0.5 μg ml−1αFas with 50 μg of CHX or 1 μg ml−1of TRAIL alone. After 0, 15 and 60 min, cells were washed with PBS and lysed. Cell lysates were immunoprecipitated with anti-caspase-8 antibody, followed by WB analysis using anti-FADD, anti-Casp10, anti-Casp8 and anti-FLIP antibodies. Control IgG was used as a negative control. Figure 2: MKRN1 depletion facilitates caspase-8 cleavage upon DR activation by causing rapid assembly of the DISC complex. ( a , b ) HeLa cells, transfected with the indicated siRNAs, were treated with 50 ng ml −1 of αFas and 5 μg ml −1 of CHX ( a ) or 50 ng ml −1 of TRAIL ( b ) for 1–3 h as indicated. Lysates were immunoblotted with anti-Casp8 and anti-Casp3 antibodies. ( c , d ) HeLa cells, transfected with siRNAs, were harvested using trypsin at 48 h post transfection. Cells were resuspended in 1 ml of complete media and treated with 0.5 μg ml −1 αFas with 50 μg of CHX or 1 μg ml −1 of TRAIL alone. After 0, 15 and 60 min, cells were washed with PBS and lysed. Cell lysates were immunoprecipitated with anti-caspase-8 antibody, followed by WB analysis using anti-FADD, anti-Casp10, anti-Casp8 and anti-FLIP antibodies. Control IgG was used as a negative control. Full size image As tumour necrosis factor-α (TNFα) also triggers extrinsic apoptosis via complex II, which is similar to the DISC complex and which consists of caspase-8, FADD and RIP1 (refs 28 , 29 ), we examined TNFα-triggered extrinsic apoptosis upon MKRN1 depletion. Similar to the above results, MKRN1 depletion facilitated caspase activation, cell death and morphological changes upon TNFα treatment ( Supplementary Fig. S7a–d ). TNFα-mediated apoptosis facilitated by MKRN1 depletion was also abolished by treatment of cells with a caspase-8 inhibitor ( Supplementary Fig. S7b ). In addition, complex II formation was enhanced upon TNFα stimulation in MKRN1-depleted cells ( Supplementary Fig. S7e ). Together, these findings suggest that MKRN1 suppresses extrinsic apoptosis by regulating common components involved in anti-Fas-, TRAIL- and TNFα-mediated apoptosis. FADD ubiquitination and degradation is MKRN1-dependent As MKRN1 is an E3 ubiquitin ligase [24] , [26] , [27] , we next asked whether MKRN1 E3 ligase activity affected the stability of proteins involved in DISC complexes. When MKRN1 was knocked-down by siRNA or short-hairpin RNA (shRNA), MKRN1 protein was barely detected and MKRN1 messenger RNA levels were reduced up to 70–80% of control mRNAs ( Fig. 3a,b ). Interestingly, we consistently observed elevated FADD protein levels without fluctuations in caspase-8 levels ( Fig. 3a ). Using quantitative reverse transcriptase PCR, we found that mRNA levels of FADD were not affected by MKRN1 depletion ( Fig. 3b ), suggesting that FADD is post-translationally regulated by MKRN1. The half-life of FADD was measured to be about 4 h based on CHX treatment. FADD breakdown was almost completely blocked by MG132, a proteasome inhibitor, but not by the lysosomal inhibitor bafilomycin A1 ( Fig. 3c ; Supplementary Fig. S8a ). Importantly, MKRN1 depletion significantly abolished FADD destabilization in a manner similar to MG132 treatment, suggesting that MKRN1 mediates the proteasomal degradation of FADD ( Fig. 3d ; Supplementary Fig. S8b ). As proteasomal degradation is largely mediated by ubiquitination, we next investigated the ubiquitination status of FADD. Endogenous ubiquitinated FADD was detectable in cells, and ubiquitination of this protein was further increased by MG132 treatment, whereas MKRN1 depletion significantly reduced FADD ubiquitination, suggesting that MKRN1 mediates FADD ubiquitination ( Fig. 3e ). Note, the levels of FADD still decrease upon CHX treatment, even with the decrease in MKRN1 protein levels ( Fig. 3c,d ). Under steady-state conditions, FADD seems to be continually turned over through ubiquitination ( Fig. 3e , lane 3). When cells are treated with CHX, these ubiquitinated FADD proteins seem to be degraded concomitantly with MKRN1 ( Fig. 3d ). We cannot exclude the possible existence of other E3 ligases that may affect FADD stability in this case. We next investigated the role of the MKRN1 depletion-induced increase in FADD expression in anti-Fas or TRAIL-mediated apoptosis by depleting FADD proteins. FADD depletion was able to rescue cells undergoing apoptosis due to MKRN1 depletion, and anti-Fas and TRAIL treatment ( Fig. 3f ). In summary, our results indicate that ablation of MKRN1 promotes FADD stabilization by abrogating FADD ubiquitination and destabilization, rendering cells susceptible to DR-mediated apoptosis. 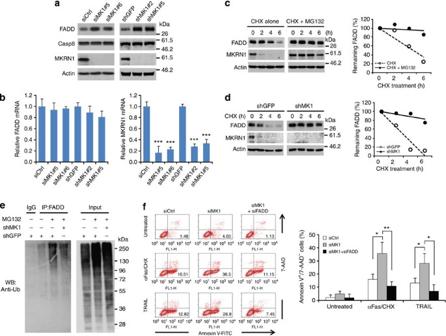Figure 3: MKRN1 knockdown induces FADD stabilization. (a) Protein levels of FADD and caspase-8 in HeLa cells transiently transfected with MKRN1 siRNA (siMK1#5 or siMK1#6) or stably expressing MKRN1 shRNA (shMK1#2 or shMK1#5) were analysed by WB. (b) Total RNA was purified from MKRN1-knockdown HeLa cells using Trizol reagent and was reverse transcribed and amplified using specific primers. The transcript levels of MKRN1 and FADD were measured by real-time PCR (data are means±s.d.;n=3, ***P<0.001 compared with siCtrl or shGFP). (c) HeLa cells were treated with 40 μg ml−1of CHX for the indicated times to determine protein stability. Cells were lysed and analysed by WB using anti-FADD and anti-MKRN1 antibodies. Representative results of three independent experiments are shown. Relative amounts of FADD were calculated after normalizing to actin, and are shown in the lower panel. (d) HeLa cells stably expressing shGFP and shMK1#2 were treated with 40 μg ml−1of CHX for the indicated times, followed by WB analysis as described above. Representative results of three independent experiments are shown. Relative amounts of FADD were calculated after normalizing to actin, and are shown in the lower panel. (e) Endogenous FADD ubiquitination upon MKRN1 ablation. Lysates from MKRN1-knockdown HeLa cells were immunoprecipitated with anti-FADD antibody followed by WB analysis using HRP-conjugated anti-Ub antibodies under denaturing conditions. For the detailed procedure, see theSupplementary Methods. (f) HeLa cells were transfected with siMK1#5 in the absence and presence of FADD siRNA for 48 h, and treated with αFas and TRAIL as described inFig. 1e. Apoptosis was measured using Annexin V and 7-AAD staining followed by flow cytometry. Representative density plot data are shown in upper panel and summarized in lower panel (data are means±s.d.;n=3, *P<0.05, **P<0.01). Figure 3: MKRN1 knockdown induces FADD stabilization. ( a ) Protein levels of FADD and caspase-8 in HeLa cells transiently transfected with MKRN1 siRNA (siMK1#5 or siMK1#6) or stably expressing MKRN1 shRNA (shMK1#2 or shMK1#5) were analysed by WB. ( b ) Total RNA was purified from MKRN1-knockdown HeLa cells using Trizol reagent and was reverse transcribed and amplified using specific primers. The transcript levels of MKRN1 and FADD were measured by real-time PCR (data are means±s.d. ; n =3, *** P <0.001 compared with siCtrl or shGFP). ( c ) HeLa cells were treated with 40 μg ml −1 of CHX for the indicated times to determine protein stability. Cells were lysed and analysed by WB using anti-FADD and anti-MKRN1 antibodies. Representative results of three independent experiments are shown. Relative amounts of FADD were calculated after normalizing to actin, and are shown in the lower panel. ( d ) HeLa cells stably expressing shGFP and shMK1#2 were treated with 40 μg ml −1 of CHX for the indicated times, followed by WB analysis as described above. Representative results of three independent experiments are shown. Relative amounts of FADD were calculated after normalizing to actin, and are shown in the lower panel. ( e ) Endogenous FADD ubiquitination upon MKRN1 ablation. Lysates from MKRN1-knockdown HeLa cells were immunoprecipitated with anti-FADD antibody followed by WB analysis using HRP-conjugated anti-Ub antibodies under denaturing conditions. For the detailed procedure, see the Supplementary Methods . ( f ) HeLa cells were transfected with siMK1#5 in the absence and presence of FADD siRNA for 48 h, and treated with αFas and TRAIL as described in Fig. 1e . Apoptosis was measured using Annexin V and 7-AAD staining followed by flow cytometry. Representative density plot data are shown in upper panel and summarized in lower panel (data are means±s.d. ; n =3, * P <0.05, ** P <0.01). Full size image The observation that FADD stability increased upon MKRN1 depletion led us to examine if FADD ubiquitination and stability are directly regulated by MKRN1. Indeed, endogenous as well as exogenous FADD and MKRN1 were able to interact with each other ( Fig. 4a ; Supplementary Fig. S9a,b ). Immunoprecipitation using deletion mutants showed that the carboxy-terminal domain of FADD (190–208 amino acids) interacts with MKRN1 ( Supplementary Fig. S9c ). Finally, we found a direct interaction between MKRN1 and FADD based on an in vitro binding assay using recombinant glutathione S -transferase (GST)-FADD and in vitro translated HA-MKRN1 ( Fig. 4b ). Consistently, increased levels of exogenous MKRN1 induced FADD destabilization ( Fig. 4c ). MG132 treatment reversed this process, suggesting the involvement of the 26S proteasome ( Fig. 4d ). As expected, FADD ubiquitination increased upon addition of MKRN1 ( Fig. 4e ). We next investigated the role of the E3 ligase activity of MKRN1 on FADD ubiquitination using the enzymatically inactive H307E MKRN1 mutant [24] , [26] , [27] . The H307E mutant failed to induce FADD ubiquitination despite its ability to bind to FADD ( Fig. 4f ; Supplementary Fig. S9d ). CHX treatment revealed that MKRN1 H307E did not affect the half-life of the FADD protein, whereas WT MKRN1 reduced the half-life of FADD ( Fig. 4g ). Furthermore, H307E failed to degrade FADD in contrast to WT MKRN1 ( Fig. 4h ), indicating the critical roles of the MKRN1 ring domain in FADD ubiquitination and degradation. 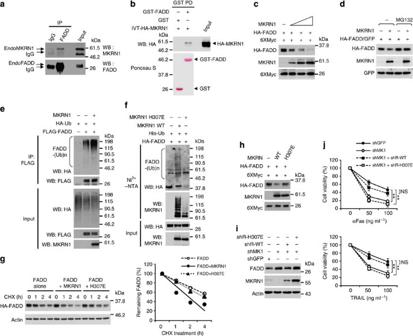Figure 4: MKRN1 suppresses extrinsic apoptosis by mediating FADD degradation. (a) The interaction between endogenous MKRN1 and endogenous FADD in HeLa cells was demonstrated by immunoprecipitation–WB analyses. (b) A direct interaction between MKRN1 and FADD was tested using bacterially purified GST-FADD andin vitrotranslated HA-MKRN1. GST-FADD was incubated with HA-MKRN1 and pulled down with glutathione sepharose beads. FADD-bound MKRN1 was detected with anti-HA antibody. (c) HeLa cells were transfected with a plasmid expressing HA-FADD and increasing amounts of MKRN1. Protein levels of FADD were determined by WB analysis using anti-HA antibody. 6XMyc (approximately 20 kDa) was used as the transfection control. (d) HeLa cells, transfected with the indicated plasmid, were treated with 10 μM MG132 for 3 h. (e) HeLa cells were transfected with the indicated plasmid, treated with MG132 for 3 h and lysed in 1% SDS buffer. FLAG-FADD was purified by immunoprecipitation using an anti-FLAG antibody, followed by WB analysis using an anti-HA antibody. (f) HeLa cells were transfected with the indicated plasmid and then treated with MG132. Cells were lysed in 6 M guanidine-HCl, and ubiquitinated proteins were purified using Ni2+-NTA beads. His-purified proteins were detected by WB analysis. (g) HeLa cells were transfected with FADD in the absence or presence of MKRN1 WT or H307E for 24 h, and then treated with CHX at the indicated time points. Relative amounts of FADD were calculated after normalizing to actin, and are shown in the right panel. (h) The effect of MKRN1 H307E on FADD protein levels was tested as described in the legend forc. (i) shRNA-resistant mutant MKRN1 WT (shR-WT) or H307E (shR-H307E) was stably expressed in HeLa/shMKRN1#2 (shMK1) cells using a retroviral vector. Protein levels of FADD were determined by WB analysis. (j) The viability of HeLa/shMK1 cells transfected with shR-WT or shR-H307E after treatment with αFas and CHX or TRAIL (as described in the legend forFig. 1e) was determined using the Cell Titer Glo Luminescent Cell Viability Assay kit (data are means±s.d.;n=3, **P<0.01). Figure 4: MKRN1 suppresses extrinsic apoptosis by mediating FADD degradation. ( a ) The interaction between endogenous MKRN1 and endogenous FADD in HeLa cells was demonstrated by immunoprecipitation–WB analyses. ( b ) A direct interaction between MKRN1 and FADD was tested using bacterially purified GST-FADD and in vitro translated HA-MKRN1. GST-FADD was incubated with HA-MKRN1 and pulled down with glutathione sepharose beads. FADD-bound MKRN1 was detected with anti-HA antibody. ( c ) HeLa cells were transfected with a plasmid expressing HA-FADD and increasing amounts of MKRN1. Protein levels of FADD were determined by WB analysis using anti-HA antibody. 6XMyc (approximately 20 kDa) was used as the transfection control. ( d ) HeLa cells, transfected with the indicated plasmid, were treated with 10 μM MG132 for 3 h. ( e ) HeLa cells were transfected with the indicated plasmid, treated with MG132 for 3 h and lysed in 1% SDS buffer. FLAG-FADD was purified by immunoprecipitation using an anti-FLAG antibody, followed by WB analysis using an anti-HA antibody. ( f ) HeLa cells were transfected with the indicated plasmid and then treated with MG132. Cells were lysed in 6 M guanidine-HCl, and ubiquitinated proteins were purified using Ni 2+ -NTA beads. His-purified proteins were detected by WB analysis. ( g ) HeLa cells were transfected with FADD in the absence or presence of MKRN1 WT or H307E for 24 h, and then treated with CHX at the indicated time points. Relative amounts of FADD were calculated after normalizing to actin, and are shown in the right panel. ( h ) The effect of MKRN1 H307E on FADD protein levels was tested as described in the legend for c . ( i ) shRNA-resistant mutant MKRN1 WT (shR-WT) or H307E (shR-H307E) was stably expressed in HeLa/shMKRN1#2 (shMK1) cells using a retroviral vector. Protein levels of FADD were determined by WB analysis. ( j ) The viability of HeLa/shMK1 cells transfected with shR-WT or shR-H307E after treatment with αFas and CHX or TRAIL (as described in the legend for Fig. 1e ) was determined using the Cell Titer Glo Luminescent Cell Viability Assay kit (data are means±s.d. ; n =3, ** P <0.01). Full size image We next tested whether reintroduction of shRNA-resistant WT MKRN1 (shR-WT) into MKRN1-depleted cells could prevent anti-Fas or TRAIL-induced apoptotic cell death. Elevated protein levels of endogenous FADD in MKRN1-depleted cells were reduced by ectopic expression of shR-WT but not by the shRNA-resistant MKRN1 H307E mutant (shR-H307E) ( Fig. 4i ). Furthermore, reconstitution of shR-WT in MKRN1-depleted cells suppressed caspase-8 and caspase-3 cleavage, while shR-H307E did not ( Supplementary Fig. S10 ). Finally, shR-WT, but not shR-H307E, increased the cell viability of MKRN1-knockdown cells upon anti-Fas and TRAIL treatment ( Fig. 4j ). Collectively, our data indicate that MKRN1 negatively regulates DR-mediated apoptosis by mediating FADD ubiquitination and degradation. MKRN1 depletion facilitates necrosome formation Several recent studies have indicated that the DR complex also has key roles in programmed necrosis or necroptosis, which is induced upon caspase inhibition in the presence of RIP3 [31] , [32] , [33] , [34] , [35] , [36] , [37] , [38] . As MKRN1 affects the formation of DR complexes, we investigated its involvement in necrotic cell death. We employed L929 mouse fibroblasts for this necroptosis study. Treatment of control cells with z-VAD-fmk with or without mTNFα resulted in cell death, as reported previously [31] , [39] , [40] , [41] , [42] ( Fig. 5a–c ; Supplementary Fig. S11 ). MKRN1 knockdown significantly enhanced necroptotic cell death in this cell line, and this was abrogated by treatment of cells with nec-1 ( Fig. 5a–c ). Consistent with these results, RIP1–RIP3–FADD complex formation increased upon mTNFα and z-VAD-fmk treatment under MKRN1 depletion ( Fig. 5d ). We also employed the HT-29 human colon cancer cell line, which expresses RIP3 proteins and undergoes necroptosis [31] . Unlike L929 cells, TNF or zVAD alone was not sufficient to induce cell death in HT-29 cells ( Supplementary Fig. S12a,b ). Rather, the combination of CHX and TNF (T/C), or that of z-VAD-fmk and TNF/CHX (T/C/Z), induced apoptotic or necroptotic cell death, respectively ( Supplementary Fig. S12a,b ). We observed that upon T/C treatment, MKRN1 depletion promoted apoptosis that was not blocked by nec-1 ( Supplementary Fig. S12c–e ). While HT-29/shGFP cells showed modest cell death upon treatment with T/C/Z, extensive death of HT-29/shMKRN1 cells occurred upon T/C/Z treatment due to necroptosis, as nec-1 mostly eliminated such cell death ( Supplementary Fig. S12c–e ). Furthermore, rapid formation of FADD–RIP1–RIP3 complexes was observed in HT-29/shMKRN1 cells in response to necroptotic stimuli, and the level of FADD protein in these cells was increased relative to control cells ( Supplementary Fig. S12f ). Collectively, these data suggest that when the apoptotic pathway is suppressed, MKRN1 depletion facilitates necroptosis by increasing necrosome complex formation. 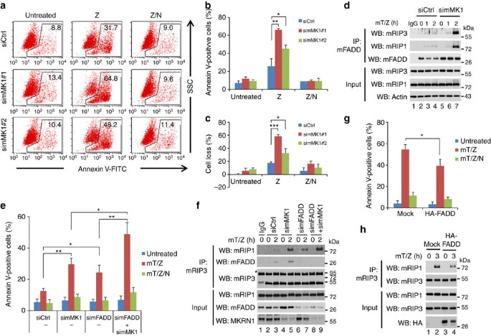Figure 5: MKRN1 knockdown enhances necroptosis in a FADD-independent manner. (a,b) L929 cells were transfected with 50 nM of control siRNA (siCtrl) or mouse MKRN1 siRNA (simMK1#1 and simMK1#2) for 48 h. Cells were treated with 20 μM of z-VAD-fmk (Z) with or without 30 μM of Nec-1 (N) for an additional 18 h. Cells undergoing necroptosis were detected by Annexin V staining and the results were confirmed by Nec-1 treatment. The mean percentages of Annexin V-positive cells from three independent experiments are shown inb. Representative dot plot data are presented ina. (c) L929 cells, transfected with the indicated siRNAs and treated as ina. Cell death was determined by measuring intracellular ATP levels using the Cell Titer Glo Luminescent Cell Viability Assay kit. (d) L929 cells were transfected with the siRNAs and treated with 5 ng ml−1of mouse TNFα (mT) and 10 μM of z-VAD-fmk (Z) for the indicated time. Cell lysates were immunoprecipitated with anti-mFADD antibody, followed by WB analysis as indicated. (e) L929 cells were transfected with the combination of 30 nM simMK1#1 and mouse FADD siRNA pool (simFADD) as indicated. Control siRNA was used to keep the siRNA concentration to 60 nM. Cells were treated with mT/Z with or without 30 μM of Nec-1 (N) for 3 h. Necroptotic cells were detected as described inaandb. (f) L929 cells, transfected the indicated siRNAs, were treated with mT/Z. Cell lysates were immunoprecipitated with anti-mRIP3 antibody, followed by WB analysis as indicated. (g) L929 cells were transfected with a plasmid expressing HA-FADD and treated for 4 h as indicated. Necroptotic cells were detected as described ina. The mean percentages of Annexin V-positive cells from three independent experiments are shown ing. Representative dot plot data are presented inSupplementary Fig. S14b. (h) L929 cells, transfected with the plasmid expressing HA-FADD, were treated with mT/Z. RIP1–RIP3 complexes were detected as described above. All bars represent the mean values±s.d.;n=3, *P<0.05, **P<0.01, ***P<0.001. Figure 5: MKRN1 knockdown enhances necroptosis in a FADD-independent manner. ( a , b ) L929 cells were transfected with 50 nM of control siRNA (siCtrl) or mouse MKRN1 siRNA (simMK1#1 and simMK1#2) for 48 h. Cells were treated with 20 μM of z-VAD-fmk (Z) with or without 30 μM of Nec-1 (N) for an additional 18 h. Cells undergoing necroptosis were detected by Annexin V staining and the results were confirmed by Nec-1 treatment. The mean percentages of Annexin V-positive cells from three independent experiments are shown in b . Representative dot plot data are presented in a . ( c ) L929 cells, transfected with the indicated siRNAs and treated as in a . Cell death was determined by measuring intracellular ATP levels using the Cell Titer Glo Luminescent Cell Viability Assay kit. ( d ) L929 cells were transfected with the siRNAs and treated with 5 ng ml −1 of mouse TNFα (mT) and 10 μM of z-VAD-fmk (Z) for the indicated time. Cell lysates were immunoprecipitated with anti-mFADD antibody, followed by WB analysis as indicated. ( e ) L929 cells were transfected with the combination of 30 nM simMK1#1 and mouse FADD siRNA pool (simFADD) as indicated. Control siRNA was used to keep the siRNA concentration to 60 nM. Cells were treated with mT/Z with or without 30 μM of Nec-1 (N) for 3 h. Necroptotic cells were detected as described in a and b . ( f ) L929 cells, transfected the indicated siRNAs, were treated with mT/Z. Cell lysates were immunoprecipitated with anti-mRIP3 antibody, followed by WB analysis as indicated. ( g ) L929 cells were transfected with a plasmid expressing HA-FADD and treated for 4 h as indicated. Necroptotic cells were detected as described in a . The mean percentages of Annexin V-positive cells from three independent experiments are shown in g . Representative dot plot data are presented in Supplementary Fig. S14b . ( h ) L929 cells, transfected with the plasmid expressing HA-FADD, were treated with mT/Z. RIP1–RIP3 complexes were detected as described above. All bars represent the mean values±s.d. ; n =3, * P <0.05, ** P <0.01, *** P <0.001. Full size image FADD stabilization upon MKRN1 depletion prevents necroptosis Although FADD is found in the necrosome complex and is regarded as an adaptor protein that links DRs to the RIP1–RIP3 complex [9] , [31] , [32] , [42] , it appears to function as a negative regulator of necroptosis under various conditions [5] , [7] , [10] , [11] , [43] . To determine the exact function of FADD in necrosome formation in relation to MKRN1, we first depleted FADD in L929 and HT-29 cells. Consistent with a previous report [44] , knockdown of FADD significantly induced necroptosis in both cell types ( Fig. 5e ; Supplementary Fig. S13 ). Interestingly, FADD depletion resulted in a noticeable increase in RIP1–RIP3 complex formation compared with control cells, suggesting that FADD might interfere with RIP1–RIP3 complex formation ( Fig. 5f , lanes 3,7; Supplementary Fig. S13c ). To further ascertain the negative roles of FADD in necroptosis and necrosome formation, we employed L929 cells ectopically expressing HA-FADD protein. As expected, necroptosis and RIP1–RIP3 complex formation were suppressed in FADD-overexpressing cells compared with control cells ( Fig. 5g,h ; Supplementary Fig. S14 ). Based on the observation of increased necroptosis and FADD–RIP1–RIP3 complex formation upon MKRN1 depletion and the inhibitory roles of FADD on necroptosis, we hypothesized that the increase in FADD levels upon MKRN1 knockdown might restrain necroptosis. As expected, FADD knockdown in MKRN1-depleted cells further increased necroptotic cell death ( Fig. 5e ; Supplementary Fig. S13b,d ). Consistently, RIP1–RIP3 complex formation appeared to be maximized in MKRN1 and FADD-depleted cells compared with MKRN1-depleted cells ( Fig. 5f , lanes 5,9; Supplementary Fig. S13c ). Interestingly, MKRN1 depletion increased necrosome formation and necroptosis even with FADD knockdown; this suggests that MKRN1 has an as yet undefined function in regulating necroptosis independent of FADD ( Fig. 5e,f , lanes 7,9; Supplementary Fig. S13b,c ). As MKRN1 depletion only affected the stability of FADD, but not that of RIP1 or RIP3, future studies should identify MKRN1 targets other than FADD in necroptotic pathways ( Supplementary Fig. S12a ). Overall, these data suggest that MKRN1 knockdown enhances necroptosis in a FADD-independent manner, but FADD stabilization upon MKRN1 knockdown could retard necroptosis. MKRN1 inversely correlates with FADD in breast cancers To further investigate the physiological relevance of MKRN1 regulation of FADD, we assessed the expression levels of MKRN1 in various normal and cancer cells. Most breast cancer cell lines expressed high levels of MKRN1. In contrast, MCF10A, a normal mammary epithelial cell line, expressed very low levels of MKRN1 compared with the other cell lines examined ( Supplementary Fig. S15a ). An inverse correlation between the levels of MKRN1 and FADD was observed in all breast cancer cell lines with the exception of MCF10A ( Supplementary Fig. S15a–c ). We further observed that mRNA levels of MKRN1 were significantly increased in breast and cervical cancer tissues compared with those in corresponding normal tissues based on an analysis of the Oncomine database ( www.oncomine.org ) [45] ( Fig. 6a ) [46] , [47] . Investigation of breast and cervical cancer tissues in the Human Protein Atlas Database also revealed that MKRN1 protein levels in these cancer tissues were elevated compared with MKRN1 levels in normal tissues ( www.proteinatlas.org/ENSG00000133606 . 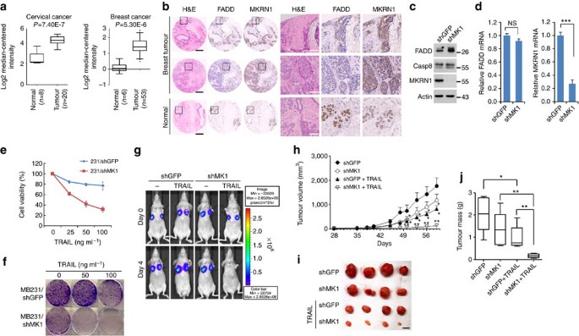Figure 6: MKRN1 is overexpressed in breast cancer and downregulation of MKRN1 suppresses tumour growth upon TRAIL treatment. (a) Expression of MKRN1 in breast and cervical cancer. Data were obtained from the Oncomine Database46,47and re-analysed. (b) Expression of MKRN1 and FADD in human breast tumours and normal tissue were examined by immunohistochemical analysis of a tissue array (Superbiochips Laboratories, Seoul, South Korea), which was stained with human MKRN1 and FADD antibodies. Representative slides of a human breast tissue arrays are shown, and the areas within the black squares are enlarged and presented in the right-side panels. Black scale bars, 0.5 mm and white scale bars, 100 μm. (c,d) Protein levels (c) and mRNA levels (d) of FADD and caspase-8 in MDA-MB-231-luc cells stably expressing shGFP or shMKRN1 were measured by WB and quantitative reverse transcriptase PCR (data are means±s.d.;n=3, ***P<0.001, NS; non-specific). (e) MDA-MB-231-luc cells expressing shGFP or shMKRN1 were treated with TRAIL for 12 h, and then cell viability was determined using the MTT assay (data are means±s.d.;n=3). (f) Cells were treated with TRAIL for 12 h and replated into 6-well plates. After 2 weeks, cells were stained with crystal violet. (g) MDA-MB-231-luc cells expressing shGFP or shMKRN1 were injected into the mammary fat pads of nude mice. At 1 week after inoculation, mice were treated with 100 μg of TRAIL by i.v. injection for 4 days. Tumours were detected by bioluminescence using the Xenogen IVIS 2000 system. Representative mice are shown in the figure (n=3). (h–j) Mice xenografted with MDA-MB-231/shMKRN1 cells were treated with 100 μg TRAIL by i.p. injection (daily, 5 days per week, 2 weeks). Tumour growth is shown in the graph (h) (data are means±s.d.;n=6, **P<0.01 between shMK1 and shMK1+TRAIL, *P<0.05 between shGFP and shGFP+TRAIL), and tumours are shown in (i). Bars, 1 cm. Tumour mass is summarized in (j) (Data are means±s.d.;n=6, **P<0.01, *P<0.01). Figure 6: MKRN1 is overexpressed in breast cancer and downregulation of MKRN1 suppresses tumour growth upon TRAIL treatment. ( a ) Expression of MKRN1 in breast and cervical cancer. Data were obtained from the Oncomine Database [46] , [47] and re-analysed. ( b ) Expression of MKRN1 and FADD in human breast tumours and normal tissue were examined by immunohistochemical analysis of a tissue array (Superbiochips Laboratories, Seoul, South Korea), which was stained with human MKRN1 and FADD antibodies. Representative slides of a human breast tissue arrays are shown, and the areas within the black squares are enlarged and presented in the right-side panels. Black scale bars, 0.5 mm and white scale bars, 100 μm. ( c , d ) Protein levels ( c ) and mRNA levels ( d ) of FADD and caspase-8 in MDA-MB-231-luc cells stably expressing shGFP or shMKRN1 were measured by WB and quantitative reverse transcriptase PCR (data are means±s.d. ; n =3, *** P <0.001, NS; non-specific). ( e ) MDA-MB-231-luc cells expressing shGFP or shMKRN1 were treated with TRAIL for 12 h, and then cell viability was determined using the MTT assay (data are means±s.d. ; n =3). ( f ) Cells were treated with TRAIL for 12 h and replated into 6-well plates. After 2 weeks, cells were stained with crystal violet. ( g ) MDA-MB-231-luc cells expressing shGFP or shMKRN1 were injected into the mammary fat pads of nude mice. At 1 week after inoculation, mice were treated with 100 μg of TRAIL by i.v. injection for 4 days. Tumours were detected by bioluminescence using the Xenogen IVIS 2000 system. Representative mice are shown in the figure ( n =3). ( h – j ) Mice xenografted with MDA-MB-231/shMKRN1 cells were treated with 100 μg TRAIL by i.p. injection (daily, 5 days per week, 2 weeks). Tumour growth is shown in the graph ( h ) (data are means±s.d. ; n =6, ** P <0.01 between shMK1 and shMK1+TRAIL, * P <0.05 between shGFP and shGFP+TRAIL), and tumours are shown in ( i ). Bars, 1 cm. Tumour mass is summarized in ( j ) (Data are means±s.d. ; n =6, ** P <0.01, * P <0.01). Full size image We next performed immunohistochemical (IHC) studies to evaluate the expression of MKRN1 and FADD in situ in histological grade 2 and 3 breast cancer tissues of 40 cases. MKRN1 and FADD were mainly detected in the cytoplasm of cancer cells, whereas FADD was detected in the nucleus in some cases. MKRN1 was expressed in 34 out of 40 breast cancer cases (85%), with a tendency to be more overexpressed in grade 3 than grade 2 breast cancer tissues ( P =0.093, χ 2 -test). FADD expression was also detected in 27 of 40 cases (67.5%), but FADD expression did not have a significant correlation with histological tumour grade. Interestingly, however, six cases (85.7%) among MKRN1 over-expressing grade 3 breast cancer tissues showed FADD underexpression, and this association was statistically significant ( P =0.006, χ 2 -test) ( Fig. 6b ). Overall, the IHC data from breast cancer samples suggest that the protein levels of MKRN1 and FADD tend to be reversely correlated in high histological grade breast cancers, indicating a possible role for MKRN1 as a negative regulator of FADD in vivo. MKRN1 depletion sensitizes breast tumours to TRAIL treatment The general overexpression of MKRN1 in breast cancer prompted us to ask whether the TRAIL sensitivity of breast cancer cells can be enhanced by MKRN1 depletion. We used MDA-MB-231 triple-negative breast cancer (TNBC) cells because these cells, which do not express the oestrogen receptor or progesterone receptor and do not have HER-2 amplification, are malignant, and patients with a TNBC phenotype have a poor prognosis [48] , [49] . MDA-MB-231-luc cells constitutively expressing luciferase were constructed to monitor tumour cell growth in vivo . We then established MDA-MB-231-luc cells stably expressing shMKRN1. MKRN1 knockdown in these cell lines was not sufficient to induce apoptosis unlike in HeLa cells, despite successful knockdown of MKRN1 ( Fig. 6c,d ). However, consistent with the HeLa cell experiments, MKRN1 depletion in MDA-MB-231-luc cells resulted in increased FADD protein levels ( Fig. 6c,d ). TRAIL treatment of MDA-MB-231/shMKRN1 cells facilitated cell death compared with that in control cells ( Fig. 6e ). Consistent with these results, depletion of MKRN1 reduced the long-term survival of TNBC cells upon TRAIL treatment ( Fig. 6f ). To further investigate the in vivo relationship between MKRN1 and TRAIL, we used an orthotropic mammary xenograft tumour model and MDA-MB-231-luc cells expressing shGFP or shMKRN1. At 1 week after implantation, mice were treated with TRAIL. Administration of TRAIL by intravenous (i.v.) injection for 4 days in MDA-MB-231/shGFP xenografts resulted in no significant change in the bioluminescence signal, whereas MDA-MB-231/shMKRN1 xenografts largely lost their bioluminescence signal after TRAIL treatment ( Fig. 6g ). Next, we prepared another sets of mice as above, then treated them with TRAIL by intraperitoneal (i.p.) injection for 5 days a week for 2 weeks and monitored tumour growth. Xenografted tumours containing cells stably transfected with shGFP grew steadily up to 1,700 mm 3 , while TRAIL treatment reduced the tumour size to 800 mm 3 . Xenografted tumours expressing shMKRN1 were 66% of the size of the tumours expressing shGFP ( Fig. 6h–j ). In contrast, the tumours of mice xenografted with cells stably expressing shMKRN1 followed by TRAIL treatment exhibited little growth, suggesting that TRAIL and MKRN1 knockdown had a synergistic negative effect ( Fig. 6h–j ). We next asked whether the effects of MKRN1 on TRAIL sensitization were associated with FADD. FADD ablation completely abrogated TRAIL-mediated caspase-8 activation and cell death in MKRN1-ablated MDA-MB-231 cells ( Fig. 7a,b ; Supplementary Fig. S16 ). When we performed xenograft assays using MDA-MB-231 expressing shMKRN1 with or without shFADD, we found that tumours expressing shMKRN1 were more sensitive to TRAIL treatment than tumours simultaneously depleted of MKRN1 and FADD, which were fairly resistant to TRAIL treatment ( Fig. 7c–e ). Taken together, these data support the hypothesis that suppression of MKRN1 in breast cancer cells increases the sensitivity of these cells to TRAIL-mediated tumour suppression in a FADD-dependent manner. 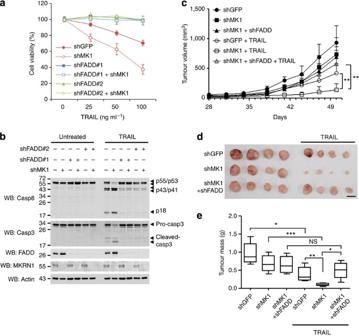Figure 7: Sensitization of TRAIL-mediated tumour suppression upon MKRN1 knockdown is abrogated by FADD depletion. (a) MDA-MB-231-luc cells stably expressing the indicated shRNAs were treated with the indicated concentration of TRAIL for 6 h, and cell viability was determined using the Cell Titer Glo Luminescent Cell Viability Assay kit (data are means±s.d.;n=3). (b) MDA-MB-231-luc cells stably expressing the indicated shRNAs were treated with 100 ng ml−1TRAIL for 3 h. Caspase-8 and -3 cleavage was measured by WB analysis. (c–e) MDA-MB-231-luc cells expressing shGFP, shMKRN1 or shFADD+shMKRN1 were injected into the mammary fat pads of nude mice. At 1 week after inoculation, mice were treated with 100 μg of TRAIL by i.p. injection (daily, 5 days per week, 2 weeks). Tumour growth is shown in the graph (c) (data are means±s.d.;n=6, **P<0.01), and tumours are shown in (d). Bars, 1 cm. Tumour mass is summarized in (e) (data are means±s.d.;n=6, *P<0.05, **P<0.01, ***P<0.001). Figure 7: Sensitization of TRAIL-mediated tumour suppression upon MKRN1 knockdown is abrogated by FADD depletion. ( a ) MDA-MB-231-luc cells stably expressing the indicated shRNAs were treated with the indicated concentration of TRAIL for 6 h, and cell viability was determined using the Cell Titer Glo Luminescent Cell Viability Assay kit (data are means±s.d. ; n =3). ( b ) MDA-MB-231-luc cells stably expressing the indicated shRNAs were treated with 100 ng ml −1 TRAIL for 3 h. Caspase-8 and -3 cleavage was measured by WB analysis. ( c – e ) MDA-MB-231-luc cells expressing shGFP, shMKRN1 or shFADD+shMKRN1 were injected into the mammary fat pads of nude mice. At 1 week after inoculation, mice were treated with 100 μg of TRAIL by i.p. injection (daily, 5 days per week, 2 weeks). Tumour growth is shown in the graph ( c ) (data are means±s.d. ; n =6, ** P <0.01), and tumours are shown in ( d ). Bars, 1 cm. Tumour mass is summarized in ( e ) (data are means±s.d. ; n =6, * P <0.05, ** P <0.01, *** P <0.001). Full size image Here, we report for the first time that FADD protein stability is regulated by the ubiquitin-proteasome pathway via the E3 ubiquitin ligase MKRN1. Various biochemical analyses, including ubiquitination and degradation assays, clearly indicated that MKRN1 targets FADD as a substrate. FADD protein levels increased under MKRN1 depletion, leading to enhanced formation of DISC complexes or complex II, extensive caspase-8 activation and subsequent extrinsic apoptosis. Based on these observations, we propose a model of how MKRN1-mediated regulation of FADD is involved in extrinsic apoptosis. In cells expressing endogenous MKRN1, FADD protein is likely maintained at moderate or low levels through MKRN1-mediated ubiquitination and degradation, possibly to protect cells from undergoing unnecessary and detrimental cell death. Upon DR activation via a death ligand, drastic cell death is still limited by the presence of MKRN1. However, cell death is likely to increase as the duration of DR activation increases. These processes are accelerated under MKRN1 depletion and the subsequent stabilization of FADD ( Fig. 2 ). We further hypothesize that the presence of endogenous MKRN1 could prevent overstimulation or overkill of cells sensitized to death ligands by delaying the activation of the cell death pathway. Our observation that various cell lines depleted of MKRN1 underwent extrinsic apoptotic cell death even without proper ligand treatment highlights the importance of maintaining FADD molecules at low levels by post-translational modification to prevent overkill ( Fig. 1 ). While MKRN1 appears to have a role in inhibiting excessive killing of normal cells, it is also plausible that the overexpression of endogenous MKRN1 could contribute to the development of cancers. For example, we found that MKRN1 was overexpressed in cervical and breast tumour tissues; this might trigger cells to undergo tumourigenesis by desensitizing cells to DR-dependent cell death ( Figs 6 and 7 ). Furthermore, our IHC analysis of a breast cancer tissue array indicated that levels of MKRN1 and FADD may be correlated. The clinical implications of these findings need to be confirmed in future studies using more breast cancer samples. In dissecting the role of FADD in the cell death pathway, we were not able to exclude the role of FADD in necroptosis. The embryonic lethality of FADD- or caspase-8-null mice complemented by RIP1- or RIP3-knockout established that RIP1 and RIP3 are both required for necroptosis [6] , [9] , [11] . When caspase-8 is inhibited by inhibitors or removal of FADD, cells undergo necroptosis via RIP1–RIP3 complex formation and the activation of downstream pathways [34] , [36] , [50] . MKRN1 depletion induced an increase in FADD–RIP1–RIP3 complex formation and resulted in more efficient necroptoptic cell death ( Fig. 5 ). Interestingly, FADD depletion concomitant with MKRN1 knockdown led to even more enhanced RIP1–RIP3 complex formation and necroptosis in both L929 and HT-29 cell lines, while overexpression of FADD restricted both processes. These findings indicate that FADD has a negative effect on necrosome formation. An additional noteworthy observation is that MKRN1 is involved, directly or indirectly, in regulating RIP1–RIP3 complex formation independent of FADD. While MKRN1 knockdown had no significant effects on either RIP1 or RIP3 protein levels, the increase in RIP1–RIP3 complex formation even with stabilized FADD under these conditions indicates that MKRN1 might regulate necroptosis by an uncharacterized pathway. Further studies are required to investigate this hypothesis. Although TRAIL is considered a good candidate drug for cancer treatment because of its low toxicity, several cancer types are resistant to TRAIL [19] , [29] , [48] , [51] , [52] . As MKRN1 modulates TRAIL sensitivity, we employed various cancer cell lines, including breast, colon and lung cancer cell lines, to investigate if there was a correlation between TRAIL sensitivity and MKRN1 expression. Most TRAIL-resistant cells, such as MCF-7, T47D, MDA-MB-468, A549 and RKO, expressed relatively higher levels of MKRN1 protein while TRAIL-sensitive cells, namely JIMT, MDA-MB-231, H460 and SW480, expressed comparably lower amounts of MKRN1 ( Supplementary Fig. S15 ). Some TRAIL-sensitive cell lines, such as Hs578T and HCT116, however, expressed high levels of MKRN1 and low levels of FADD ( Supplementary Fig. S15 ). These results suggest that while MKRN1 might contribute to TRAIL insensitivity by downregulating FADD, other factors are also likely to be involved. Based on the above results, we performed orthotropic xenograft assays using MDA-MB-231 TNBC cells. The observation that MKRN1 depletion could effectively sensitize xenografted tumours to TRAIL therapy indicates that MKRN1-related pathways are plausible, novel therapeutic targets. Regulation of MKRN1 pathways could potentially be combined with TRAIL therapy to increase the effectiveness of TRAIL therapy. Plasmids All MKRN1 constructs (pcDNA3.1-MKRN1 WT/H307E, pcDNA3-HA-MKRN1 WT/H307E, pcDNA3-FLAG-MKRN1 WT/H307E) were described previously [24] . pcDNA3-His-Ub was kindly provided by D.P. Lane [53] . pHM6-HA-Ub has been described previously [54] . pEGFP-C2 (Clontech, San Diego, CA, USA) and pCS3-MT-6XMyc vectors were used as transfection controls. HA-FADD was kindly provided by S.Y. Lee (Ewha Woman's University) and was subcloned into pcDNA3-Flag and pGEX-4T-1. Cell culture and transfection HeLa (cervical cancer cell line), H1299 (human lung carcinoma cell line), U2OS (osteosarcoma cell line), HT-29 (human colon cancer cell line), L929 (mouse fibroblast), MDA-MB-231, MDA-MB-468, MCF-7 and Hs578T (breast cancer cell lines) were maintained in DMEM supplemented with 10% fetal bovine serum (Gibco) and 1% penicillin/streptomycin (Invitrogen, Carlsbad, CA, USA) in 5% CO 2 at 37 °C. SK-BR-3, ZR-75-1 and T47D cells were maintained in RPMI with 10% fetal bovine serum and antibiotics (Gibco). HCT116 p53+/+ and p53−/− cells were kindly provided by Dr B Vogelstein (Johns Hopkins University, Baltimore, MD, USA) and were maintained in McCoy's 5A medium supplemented with 10% fetal bovine serum and antibiotics. Antibodies and chemicals The following antibodies were used for WB: FADD (610399; BD Transduction Laboratories, 1:1,000 or sc-5559; Santa Cruz, 1:500), FADD (05-486 for mouse FADD; Millipore, 1:2,000), Fas (sc-715; Santa Cruz, 1:500), Caspase-8 (9746; Cell Signaling, 1:2,000 in 5% BSA or sc-6136; Santa Cruz, 1:500), Caspase-9 (9502; Cell Signaling, 1:1,000), Caspase-10 (M059-3; MBL, 1:1,000), Caspase-3 (9662; Cell Signaling, 1:1,000), PARP (9542; Cell Signaling, 1:2,000), FLIP (NF6, ALX-804-428, Enzo, 1:1,000), RIP1 (610409; BD Transduction Laboratories, 1:1,000), hRIP3 (PA1-41533; Pierce, 1:2,000), mRIP3 (IMG-5523; Imgenex, 1:2,000), MKRN1 (A300-990A; Bethyl Laboratories, 1:2,000), HRP-conjugated-α-Ub FK2 (PW0150; Biomol, 1:1,000), HA (sc-7392 mouse; Santa Cruz, 1:1,000, sc-805 rabbit; Santa Cruz, 1:1,000, 3F10 rat; Roche, 1:3,000), FLAG (F3165 mouse; Sigma, 1:5,000, F7425 rabbit; Sigma, 1:2,000), GST (sc-138; Santa Cruz, 1:1,000), GFP (sc-8334; Santa Cruz, 1:500) and β-actin (A5316; Sigma, 1:5,000). Propidium iodide (PI; P4170), cycloheximide (CHX, C4859), trypan blue (T8154), N-ethylmaleimide (NEM, E3876), Bafilomycin A1 (B1793) and DMSO were purchased from Sigma-Aldrich. Annexin V-FITC (556547) was purchased from BD Bioscience, and 7-AAD was obtained from eBioscience. z-VAD-fmk (627610), caspase-8 inhibitor (z-IETD-fmk, 218759) and caspase-9 inhibitor (z-LEHD-fmk, 218761) were purchased from Calbiochem (San Diego, CA, USA). z-VAD-fmk was purchased from Sigma (Z116) or Imgenex (Imi-2310). Necrostatin-1 (BML-AP309) was purchased from Enzo Life Science. MG132 was purchased from A.G. Scientific, human recombinant TNF alpha (T0157) from Sigma, mouse recombinant TNF alpha from eBioscience (14-8321-62), anti-human Fas (αFas) activating antibody (05-201, CH11) from Millipore, anti-mouse Fas mAb (clone Jo2, 554254) from BD Bioscience, and His-tagged recombinant human TRAIL (Killer TRAIL, ALX-201-073) from Enzo Life. pQE-His-TRAIL was a kind gift from SH Kim (Korea National Cancer Center) and was used for the purification of His-tagged human TRAIL and for the in vivo experiments as reported previously [55] . Cell viability analysis and crystal violet staining To determine cell viability, cells were incubated with Cell Titer Glo reagent and analysed with a luminometer according to the manufacturer's protocol (Cell Titer Glo Luminescent Cell Viability Assay kit, G7571, Promega). Alternatively, cell death was measured by treating cells with MTT (1-(4,5-dimethyl-2-thiazolyl)-3,5-diphenylformazan) for 3 h. Supernatants were gently removed, and MTT formazan crystals were dissolved in DMSO and analysed using an ELISA plate reader at a wavelength of 570 nm. For crystal violet staining, cells were plated into 6-well culture dishes, fixed in 0.1% glutaraldehyde (G6257, Sigma), and stained with crystal violet 14 days after replating. Fluorescence-activated cell sorting (FACS) analysis For PI staining, cells were fixed in 70% ethanol and incubated in 40 μg ml −1 of RNase A for 30 min, followed by incubation in 100 μg ml −1 of PI for 30 min. Cell cycle was analysed using a FACScan apparatus (BD Biosciences, NJ, USA). For Annexin V/7-AAD staining, cells were harvested using trypsin, washed with binding buffer, and incubated with Annexin V-FITC and 7-AAD for 15 min according to the manufacturer's protocol (BD Biosciences, NJ, USA). Data were analysed using CellQuest Pro software (Becton-Dickinson). Immunoprecipitation and DISC immunoprecipitation Cells were lysed in a buffer composed of 50 mM Tris–HCl (pH 7.5), 150 mM NaCl, 0.5% Triton X-100 and 1 mM EDTA containing a protease inhibitor cocktail. The cell lysates were immunoprecipitated by incubation with antibodies (1 μg) for 2 h or overnight, followed by incubation with protein G Sepharose (GE Healthcare, Buckinghamshire, UK) for 2 h. Immunoprecipitates were boiled in ×2 sample buffer for 5 min. For the DISC immunoprecipitation results presented in Supplementary Fig. S6 , cells were treated with 10 μM z-VAD-fmk 24 h after transfection and then treated with αFas (50 ng ml −1 ) and CHX (5 μg ml −1 ) or TRAIL (100 ng ml −1 ) for 0.5, 1 and 2 h. Alternatively, 5×10 6 HeLa cells transfected with siRNA were resuspended in 1 ml of complete media using trypsin, and treated with αFas (0.5 μg ml −1 ) and CHX (50 μg ml −1 ) or TRAIL (1 μg ml −1 ) for 15 and 60 min in the absence of caspase inhibitors ( Fig. 2c,d ). Cells were lysed in DISC IP buffer containing 50 mM Tris–HCl (pH 7.5), 150 mM NaCl, 1% Triton X-100, 10% glycerol and 1 mM EDTA with a proteasome inhibitor cocktail. DISC complexes were purified by IP using 1 μg of α-Fas rabbit (sc-715), α-caspase-8 goat (sc-6136) or α-FADD rabbit (sc-5559) antibodies, followed by WB analysis using α-FADD mouse (05-486; 1:2,000 or 610399; 1:1,000), α-caspase-8 mouse (#9746; 1:1,000) and α-RIP1 mouse (610409; 1:1,000) antibodies. Necrosome complexes were purified by IP using 1 μg of α-caspase-8 goat (sc-6136) or α-hRIP3 (PA1-41533) for human HT-29 cells, or α-mFADD goat (sc-6036) or α-mRIP3 (IMG-5523) for mouse L929 cells, followed by WB analysis using α-FADD mouse (05-486; 1:2,000), α-caspase-8 mouse (#9746; 1:1,000), α-RIP1 mouse (610409; 1:1,000), α-hRIP3 rabbit (PA1-41533; 1:2,000) and α-mRIP3 rabbit (IMG-5523; 1:2,000) antibodies. Normal mouse IgG (sc-2025; Santa Cruz), normal rabbit IgG (sc-2027; Santa Cruz) and normal goat IgG (sc2028; Santa Cruz) were used as negative controls. Protein purification and in vitro binding assays A DNA fragment encoding human FADD protein was inserted into a pGEX-4T-1 plasmid with GST at the amino terminus. Using this plasmid, recombinant human FADD protein was expressed in Escherichia coli and purified using glutathione sepharose 4B (GE Healthcare). GST-tagged MKRN1 was purified from bacteria transformed with pGEX-4T-1-MKRN1 using GST sepharose beads according to the manufacturer's protocol (GE Healthcare). HA-MKRN1 was produced using a TNT T7-coupled reticulocyte lysate system (Promega, L4610). In vitro translated HA-MKRN1 was incubated with GST or GST-FADD for 2 h, then glutathione sepharose was added to the mixture followed by an 1 h incubation. GST complexes were washed and eluted in 10 mM reduced glutathione. Proteins were analysed by WB analysis. In vivo ubiquitination assay The ubiquitination assay was performed as described previously [24] . Briefly, cells were lysed in 6 M guanidinium-HCl buffer (pH 8) containing 5 mM N-ethylmaleimide (Sigma-Aldrich) to prevent deubiquitination. His-ubiquitin-conjugated proteins were purified by incubation with Ni 2+ -NTA agarose beads (Qiagen), washed, eluted in sample buffer containing 200 mM imidazole and 10 mM β-mercaptoethanol, and then analysed by WB. To assess endogenous ubiquitination of FADD, cells were harvested in PBS containing 10 nM NEM and lysed in 1% SDS by boiling for 10 min. Cell lysates were diluted to 0.1% SDS by adding lysis buffer containing protease inhibitors and NEM, and immunoprecipitated with anti-FADD antibodies (sc-5559, Santa Cruz), followed by WB. Transferred proteins were denatured by soaking PVDF membranes with 6 M guanidine-HCl containing 20 mM Tris–HCl (pH 7.5), 5 mM mercaptoethanol and 1 mM PMSF for 30 min at 4 °C. Ubiquitinated FADD was detected using HRP-conjugated anti-Ub (FK2, PW0150, Biomol). An ubiquitination assay using HA-Ub was also performed by immunoprecipitation under denaturing conditions (1% SDS). Human breast cancer tissue microarray analyses Paraffin-embedded normal breast and breast cancer tissues were obtained from Superbiochips Laboratories (Seoul, South Korea). Expression levels of MKRN1 and FADD were evaluated by immunohistochemistry using anti-MKRN1 (IHC-00492, Bethyl Laboratories) and anti-FADD (610399, BD Transduction Laboratories) antibodies, respectively. Orthotropic xenograft model and in vivo TRAIL treatment Approximately 1×10 6 MDA-MB-231-luc stable cells expressing shGFP or shRNA were resuspended in 50 μl of PBS and 50 μl of Matrigel matrix (BD Sciences) and then inoculated subcutaneously into both mammary fat pads of 6-week-old female specific Balb/c nude mice (Central Lab Animal Inc., Korea). At 1 week after inoculation, mice bearing xenograft tumours were treated with 100 μg of TRAIL by i.v. injection for 4 days or by i.p. injection (daily, 5 days per week, 2 weeks). Tumour volume was measured using calipers and calculated according to the following formula: volume=length×width 2 ×0.5236. All animal experiments were performed under specific pathogen-free facilities and conditions in accordance with the Guidelines for the Care and Use of Laboratory Animals of the National Cancer Center (Korea). Statistical analyses All statistical analyses were performed by the unpaired two-tailed t -test using Prism (version 5.0; GraphPad). To assess whether differences between groups were significant in xenograft experiment, one-way ANOVA was also implemented in Prism (version 5.0; GraphPad). Information on RNA interferences, stable cell lines and reverse transcriptase PCR are provided in the Supplementary methods . How to cite this article: Lee, E.-W. et al . Ubiquitination and degradation of the FADD adaptor protein regulate death receptor-mediated apoptosis and necroptosis. Nat. Commun. 3:978 doi: 10.1038/ncomms1981 (2012).